Spontaneous transmembrane helix insertion thermodynamically mimics translocon-guided insertion The favourable transfer free energy for a transmembrane (TM) α-helix between the aqueous phase and lipid bilayer underlies the stability of membrane proteins. However, the connection between the energetics and process of membrane protein assembly by the Sec61/SecY translocon complex in vivo is not clear. Here, we directly determine the partitioning free energies of a family of designed peptides using three independent approaches: an experimental microsomal Sec61 translocon assay, a biophysical (spectroscopic) characterization of peptide insertion into hydrated planar lipid bilayer arrays, and an unbiased atomic-detail equilibrium folding-partitioning molecular dynamics simulation. Remarkably, the measured free energies of insertion are quantitatively similar for all three approaches. The molecular dynamics simulations show that TM helix insertion involves equilibrium with the membrane interface, suggesting that the interface may play a role in translocon-guided insertion. Transmembrane (TM) α-helices of proteins embedded in plasma membranes are highly enriched in amino acids with non-polar side chains, such as leucine and isoleucine. Potential TM helices in an amino-acid sequence can be identified using hydropathy plots [1] , [2] , which are based upon the sliding-window method [3] . If a true thermodynamic hydrophobicity scale is used [4] with a sliding window of about 20 amino acids, the window sum is an estimate of the free energy of transfer of an α-helix between the aqueous phase and the 30-Å-thick hydrocarbon core of the lipid bilayer (Δ G wbi , Fig. 1a ). Although this free energy is clearly relevant to the question of TM helix stability, its connection to the energetics of TM helix insertion in vivo by the Sec translocon (Δ G app , Fig. 1a ) is far from clear. Understanding the connection between Δ G wbi and Δ G app , which is the goal of the work presented here, is crucial for a quantitative description of membrane protein assembly, folding, and stability. 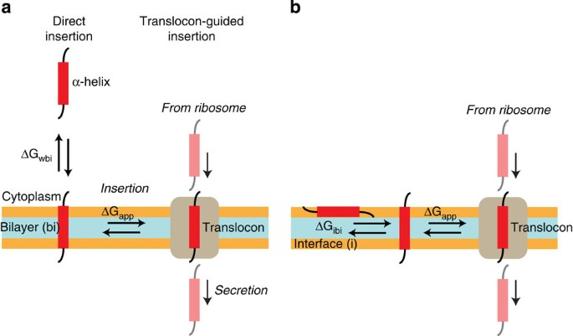Figure 1: Schematic comparisons of spontaneous transmembrane (TM) helix insertion with translocon-guided insertion. (a) The thermodynamic stability of TM helices is generally thought of as the free energy of transfer ΔGwbiof a helix from water to bilayer. Translocon-guided insertion of helices is characterized by an apparent free energy of transfer ΔGappfrom translocon to bilayer. The fundamental question addressed in this paper is the relationship between the two free-energy values. (b) All-atom equilibrium simulations presented in this paper show that helical peptides are either across the membrane (TM) or on the membrane interfaces, indicating that the actual free energy determined by the simulations ΔGibiis for transfer from the bilayer interface to TM. This figure is based on Fig. 7 of Schowet al.24 Figure 1: Schematic comparisons of spontaneous transmembrane (TM) helix insertion with translocon-guided insertion. ( a ) The thermodynamic stability of TM helices is generally thought of as the free energy of transfer Δ G wbi of a helix from water to bilayer. Translocon-guided insertion of helices is characterized by an apparent free energy of transfer Δ G app from translocon to bilayer. The fundamental question addressed in this paper is the relationship between the two free-energy values. ( b ) All-atom equilibrium simulations presented in this paper show that helical peptides are either across the membrane (TM) or on the membrane interfaces, indicating that the actual free energy determined by the simulations Δ G ibi is for transfer from the bilayer interface to TM. This figure is based on Fig. 7 of Schow et al. [24] Full size image Membrane proteins are assembled with the aid of the heterotrimeric Sec translocon, specifically Sec61αβγ in mammals and SecYEG in bacteria [5] , [6] , [7] , [8] . The SecY/Sec61 complex also guides the secretion of soluble proteins. Insertion and secretion of polypeptides occur cotranslationally in eukaryotes, as the nascent chain emerges from translocon-docked ribosomes. The Sec61 complex acts as a switch that directs sufficiently hydrophobic segments of elongating nascent chains into the membrane as TM helices while allowing more polar secreted segments to pass through the membrane into the interior of the endoplasmic reticulum (ER). The TM selection rules followed by the Sec61 complex have been determined [9] , [10] by means of an in vitro expression system supplemented with dog pancreas ER vesicles (rough microsomes) using hundreds of so-called H-segments inserted into a host protein, Escherichia coli leader peptidase [11] . The rules are described by means of apparent free energies of transfer (Δ G app ) of helices between the translocon and bilayer ( Fig. 1 ). Establishing a quantitative relationship between Δ G app and the water-to-bilayer free energy of transfer is problematic, because direct experimental determinations of Δ G wbi are rarely possible owing to aggregation of highly hydrophobic peptides in the aqueous phase [12] . Direct determinations are theoretically possible at aqueous concentrations low enough to prevent aggregation, but the concentrations required are so low as to be impractical to measure accurately in most cases. The only practical approach is to use microsecond-scale equilibrium molecular dynamics simulations, which can measure, in essence, water-to-bilayer partitioning at infinite dilution. Using this approach, Ulmschneider et al. [13] measured the partitioning of ace-L n -amide and ace-GGPG-L n -GPGG-amide peptides ( n =5 … 12) into palmitoyloleoylphosphatidycholine (POPC) bilayers and compared the resulting Δ G wbi free energies with experimental measurements [14] of Δ G app . Two important observations resulted. First, consistent with the very low aqueous solubility of hydrophobic peptides, the simulations revealed that the peptides quickly adsorbed at the membrane interface and never subsequently desorbed. The measured values of Δ G wbi thus corresponded to transfer free energies from the bilayer interface to TM orientations across the bilayer hydrocarbon core. This observation is completely consistent with extensive studies of the interfacial partitioning of peptides [2] . The second important observation was that the Δ G wbi ( n ) values exactly paralleled the Δ G app ( n ) values with a simple offset of about −2 kcal mol −1 with Δ G wbi ( n ). A fundamental question is how the observed offset would be affected by changing the polarity of the H-segment. To begin answering that question, we have altered the polarity of the segment by introducing a single arginine at the center of the polyleucine H-segment. We chose arginine for three reasons. First, the introduction of a charged residue should cause a strong perturbation of H-segment polarity. Second, Arg cannot be deprotonated when inserted into the center of a lipid bilayer based upon nuclear magnetic resonance measurements [15] and simulations [16] ; this eliminates complications that might arise from protonation–deprotonation reactions. Third, the use of Arg provided an opportunity to examine further the contentious finding of Hessa et al. [10] that the free-energy cost of inserting a single arginine into the center of a TM helix is only +2 kcal mol −1 . This small value of was contentious, because computational models predicted prohibitively large penalties of 15 kcal mol −1 or more [17] , [18] , [19] , [20] , [21] , [22] , [23] , [24] , [25] , [26] . Much of the disagreement has been due to disconnection between the quantities that the simulations and experiments actually measure. While the experimental assay measured the propensity with which the mammalian Sec61 translocon inserts 19-residue arginine-containing TM segments into the ER membrane, the computational methods calculated the free energy of burying an isolated guanidinium group in the hydrophobic core of a lipid bilayer. Attempts have been made to connect the two results via thermodynamic cycles [24] , [25] , [26] , [27] . However, accurate determination of the free-energy components of a thermodynamic cycle depends crucially on a detailed knowledge of the structural and conformational ensemble of the equilibrium states, between which the free energies are to be determined. For the translocon assay, these states are currently not known [9] , [10] , [26] , while the computational free-energy calculations are based on empirical assumptions about the nature of these states. In the experiments reported here, we used three independent approaches to examine polyleucine segments carrying a central Arg residue: (a) an experimental microsomal Sec61 translocon assay, (b) spectroscopic characterization of peptide insertion into hydrated planar lipid bilayer arrays, and (c) an unbiased atomic-detail equilibrium folding-partitioning molecular dynamics simulation. Great care was taken to design the study such that all three methods could be compared directly with each other. Direct quantification, both experimentally and computationally, of the free-energy difference (Δ G ) between two states requires that both states be measurably populated at equilibrium. In the present context, this is best achieved by designing TM segments that have partitioning free energies close to Δ G =0, so that the populations of both the inserted and non-inserted states are about equal. Because the Δ G of a peptide can only be estimated at the design stage, we chose a series of symmetric polyleucine peptides of the type G-L n RL n -G ( n =5, 6, 7, 8). Varying the number of flanking leucine residues on either side of the central arginine allowed the partitioning free energy to be modulated systematically, with longer peptides expected to insert more favourably into the lipid bilayer than shorter segments, which cannot fully span the bilayer. This allowed selection of peptides for which Δ G could be determined accurately from the inserted- and non-inserted-state populations. A polyleucine scaffold was chosen, because it forms near-perfect α-helices, thus minimizing the risk of guanidinium side chain interactions with the peptide backbone. The peptide termini were acetylated (N terminus) and amidated (C terminus) to avoid kinetic barriers that arise from having to transport charged end-groups across the hydrophobic bilayer core. Δ G from the translocon assay The insertion propensity of the peptides into the ER membrane was determined using a microsomal translocation assay [9] , [10] . Each peptide sequence was introduced as an extra H-segment into the large luminal P2 domain of the model protein leader peptidase (LepB) from E. coli . Each H-segment was flanked by GGPG– and –GPGG tetrapeptides at its N- and C termini, respectively, to ‘insulate’ the H-segment from the LepB carrier protein [9] , [10] . Glycosylation sites were placed on either side of the segment to allow quantitation of the insertion propensity. The protein was then expressed in vitro in the presence of ER-derived dog pancreas rough microsomes. Because glycosylation only takes place in the interior of the microsome, membrane-inserted segments are singly glycosylated, whereas translocated segments are doubly glycosylated. The insertion propensity P TM = f 1g /( f 1g + f 2g ) of the segment was determined by phosphoimager scans of SDS–polyacrylamide gel electrophoresis (PAGE) gels that measure the fractions of singly ( f 1g ) and doubly ( f 2g ) glycosylated proteins. As shown in Fig. 2a and Supplementary Fig. 1 , the SDS–PAGE results reveal that increasing the number of leucine residues shifts the insertion propensity from a predominantly non-inserted configuration (for L 5 RL 5 ) towards a fully inserted configuration (for L 8 RL 8 ). 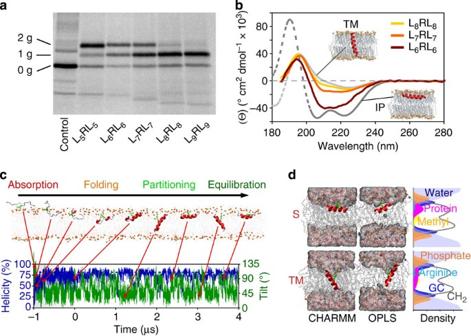Figure 2: Experimental data forin vitrotranslocon-guided insertion, orientation of synthetic peptides in POPC lipid bilayers and simulations of spontaneous insertion. (a) SDS–PAGE analysis of LepB constructs containing the GGPG-LnRLn-GPGG peptides as an added H-segment. Glycosylation sites on either side of the segment allow quantification of inserted (singly glycosylated, 1 g) and non-inserted (doubly glycosylated, 2 g) configurations. Increasing the number of leucine residues in the H-segment shifts the equilibrium from doubly to singly glycosylated peptides, with L6RL6and L7RL7showing substantial populations of both forms. Proteins that remain unglycosylated (0 g), never entered the translocon and are excluded from the measurement. The full SDS–PAGE gel is presented inSupplementary Fig. 1. (b) Oriented synchrotron radiation circular dichroism (OSRCD) spectra of the G-WLn−1RLn-G peptides in stacked POPC lipid bilayers (peptide/lipid=1/100, relative hydration=100%). Theoretical reference spectra31,32for α-helical peptides oriented parallel (TM, tilt angle≈0°) and perpendicular (IP, tilt angle≈90°) to the membrane normal (coaxial to the light beam) are shown in grey. (c) Unbiased folding-partitioning simulation of the G-L7RL7-G (L7RL7) peptide (c.f.Table 1). Absorption and interfacial folding is rapid and typically completed within 400 ns. The arginine residue, which is highlighted in green, retains contact with the lipid headgroup phosphates at all times (seeSupplementary Table 1). (d) Representative snapshots of the L7RL7peptide simulation showing the two dominant states present at equilibrium. The configurations consist of a surface (S)-adsorbed and a transmembrane (TM)-inserted helical peptide, irrespective of the force field employed. The density profiles are averages over the S and TM states of the OPLS simulation of L7RL7(tS=70 ns,tTM=130 ns). GC indicates the glycerol backbone distribution. In the TM state, the arginine residue is buried more deeply in the hydrophobic region of the bilayer. Phosphates (orange spheres) and water are frequently pulled into the bilayer to help solvate the charged guanidinium group. The Gaussian distribution of the peptide on the bilayer leaflet is noticeably broader and reaches deeper into the hydrophobic bilayer core. Figure 2: Experimental data for in vitro translocon-guided insertion, orientation of synthetic peptides in POPC lipid bilayers and simulations of spontaneous insertion. ( a ) SDS–PAGE analysis of LepB constructs containing the GGPG-L n RL n -GPGG peptides as an added H-segment. Glycosylation sites on either side of the segment allow quantification of inserted (singly glycosylated, 1 g) and non-inserted (doubly glycosylated, 2 g) configurations. Increasing the number of leucine residues in the H-segment shifts the equilibrium from doubly to singly glycosylated peptides, with L 6 RL 6 and L 7 RL 7 showing substantial populations of both forms. Proteins that remain unglycosylated (0 g), never entered the translocon and are excluded from the measurement. The full SDS–PAGE gel is presented in Supplementary Fig. 1 . ( b ) Oriented synchrotron radiation circular dichroism (OSRCD) spectra of the G-WL n −1 RL n -G peptides in stacked POPC lipid bilayers (peptide/lipid=1/100, relative hydration=100%). Theoretical reference spectra [31] , [32] for α-helical peptides oriented parallel (TM, tilt angle≈0°) and perpendicular (IP, tilt angle≈90°) to the membrane normal (coaxial to the light beam) are shown in grey. ( c ) Unbiased folding-partitioning simulation of the G-L 7 RL 7 -G (L 7 RL 7 ) peptide (c.f. Table 1 ). Absorption and interfacial folding is rapid and typically completed within 400 ns. The arginine residue, which is highlighted in green, retains contact with the lipid headgroup phosphates at all times (see Supplementary Table 1 ). ( d ) Representative snapshots of the L 7 RL 7 peptide simulation showing the two dominant states present at equilibrium. The configurations consist of a surface (S)-adsorbed and a transmembrane (TM)-inserted helical peptide, irrespective of the force field employed. The density profiles are averages over the S and TM states of the OPLS simulation of L 7 RL 7 ( t S =70 ns, t TM =130 ns). GC indicates the glycerol backbone distribution. In the TM state, the arginine residue is buried more deeply in the hydrophobic region of the bilayer. Phosphates (orange spheres) and water are frequently pulled into the bilayer to help solvate the charged guanidinium group. The Gaussian distribution of the peptide on the bilayer leaflet is noticeably broader and reaches deeper into the hydrophobic bilayer core. Full size image Δ G from synthetic peptides in oriented lipid bilayers To analyse insertion of the corresponding synthetic L n RL n peptides, the time-averaged orientation of the peptides in oriented planar lipid bilayer arrays was determined using oriented synchrotron radiation circular dichroism (OSRCD) spectroscopy. All four peptides were synthesized using solid-phase synthesis and purified using reverse-phase high-pressure liquid chromatography (see Supplementary Information ). The sequences differed from the equivalent H-segments in that the GGPG– and –GPGG insulating flanks were replaced by a single glycine, which avoids dilution of the helical circular dichroism spectrum of the L n RL n segment by the unstructured flanks (see Methods). To facilitate purification and concentration measurements, the N-terminal leucine of each peptide was replaced by a tryptophan, which has the same Δ G app as leucine in the translocon assay when near the ends of the TM helices. The validity of this approach was verified by control simulations of the GWL 6 RL 7 G peptide, which showed the insertion probability to be identical to that of the GL 7 RL 7 G peptide (see Supplementary Fig. 2 ; Table 1 ). Oriented multi-bilayer arrays were formed by depositing an organic solution containing both peptide and lipid onto quartz substrates. Highly oriented arrays form spontaneously after slow evaporation of the organic solvent followed by vapor-phase hydration at 100% relative humidity [12] , [28] , [29] . Films formed in this way typically contain stacks of ~1,000 bilayers highly aligned parallel to the quartz substrate, as determined by neutron diffraction [30] . Table 1 Summary of simulation results for polyleucine-based peptides in POPC lipid bilayers. Full size table The net orientation of the synthetic peptides inside the planar POPC bilayer stacks was determined by recording SRCD spectra with the light beam perpendicular to the quartz substrate [31] , [32] . Figure 2b shows the measured spectra together with the theoretically predicted spectra for α-helices aligned perpendicular and parallel to the bilayer normal. Spectra could only be obtained for two peptides: the spectrum of L 8 RL 8 is typical for a TM helix, while the spectra for L 7 RL 7 and L 6 RL 6 suggest that the conformational population averages contain an increasing proportion of surface-bound helical conformers. For L 6 RL 6 , P TM ≈30–50%, Δ G ≈0–0.5 kcal mol −1 ) and for L 7 RL 7 , P TM ≈70–90%, Δ G ≈−0.5 to −1.1 kcal mol −1 . The spectrum for L 5 RL 5 is atypical, with peaks at 229 nm indicative of interfacial aggregates ( Supplementary Fig. 3 ). Δ G from folding-partitioning simulations Finally, to determine computationally the free energy of peptide insertion into the membrane of glycine-flanked segments (see Methods), we used unbiased multi-microsecond atomic-detail folding-partitioning simulations at an elevated temperature of 140 °C. We have recently demonstrated that this in silico approach allows direct quantification of the transfer free energy of thermostable peptides from the equilibrium ensembles of peptide configurations in the presence of a lipid bilayer [13] , [33] , [34] . As in the synthetic implementation, the GGPG– and –GPGG insulating flanks were replaced by a single glycine, to make them identical to the synthetic implementation and to speed up partitioning kinetics, because transporting the unstructured GGPG/GPGG flanks across the hydrophobic bilayer core during TM insertion of the peptide is associated with a large energetic penalty. The removal of the flanking segments has been shown not to affect the overall partitioning free energies for a related series of polyleucine peptides [13] . At the beginning of each simulation, a single peptide was placed in bulk water about 15 Å from the surface of a POPC lipid bilayer in a completely extended configuration. The peptide was then allowed to fold freely, as well as partition spontaneously into and out of the lipid bilayer. No restraints or biasing potentials were applied. Simulation timescales of <400 ns were sufficient to capture the initial non-equilibrium bilayer absorption and folding of the peptide, while a full characterization of the structural and configurational ensemble present at equilibrium typically required several microseconds. Figure 2c summarizes this method. The non-equilibrium part of the simulations is much shorter than for globular proteins of similar size. This is because the cost of a single unpaired backbone hydrogen-bonding group in the bilayer is very large [2] (≈5 kcal mol −1 ), which drives rapid secondary structure formation. Table 1 summarizes the thermodynamic and kinetic quantities observed from the simulations. All peptides show only two states at equilibrium, with the first state (S) consisting of a surface absorbed, predominantly helical peptide tilted at an angle of ~90° with respect to the membrane normal, and the second state (TM) consisting of a TM-inserted helix with a tilt of ~30° ( Fig. 3 ). Each state is represented by a configurational and conformational ensemble ( Supplementary Fig. 4 ), which is dominated by helical conformers ( Supplementary Fig. 5 ). The bilayer responds to burial of the charged arginine side chain by localized deformation ( Supplementary Fig. 6 ), caused by tight hydrogen-bonding interactions that pull down lipid phosphate headgroups into the bilayer core ( Supplementary Table 1 ). This enables the guanidinium group to remain in contact with water even when deeply buried ( Supplementary Fig. 7 ). No bulk-phase aqueous states are sampled at equilibrium, consistent with the experimentally confirmed insolubility of the peptides. That is, only two states are observed (see Fig. 4a ): interface (S) and TM. 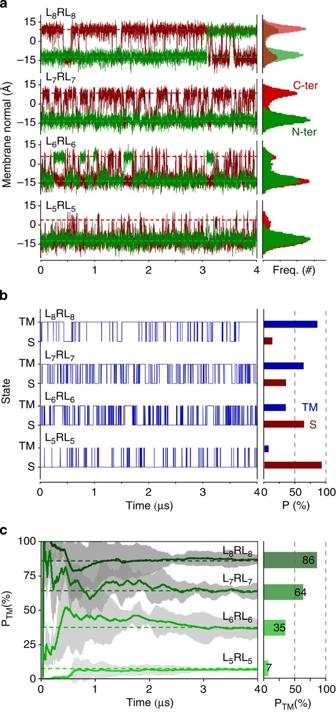Figure 3: Quantification of the kinetics and thermodynamics of peptide partitioning derived from equilibrium simulations. (a) Analysis of the positions of the peptide N termini (green) and C termini (red) along the membrane normal reveals the two-state behaviour of the system. (b) Peptides in the transmembrane (TM) state have one terminus at each of the two membrane interfaces, while peptides in the surface-bound (S) state have both termini in the same membrane interface. This allows plotting the state transitions from the analysis of the peptide termini position along the membrane normal (a). Knowledge of the state as a function of simulation time allows direct determination of the S and TM population averages, as well as analysis of state lifetimes, transition rates and related kinetics. The populations and associated free energies are given inTable 1. (c) Plots of the block-averaged TM-state propensity against the simulation time shows that the systems require at least 3 μs for full convergence. The equivalent kinetics for the L7RL7CHARMM simulation shows similar ΔG, but much slower kinetics (seeSupplementary Fig. 5). Figure 3: Quantification of the kinetics and thermodynamics of peptide partitioning derived from equilibrium simulations. ( a ) Analysis of the positions of the peptide N termini (green) and C termini (red) along the membrane normal reveals the two-state behaviour of the system. ( b ) Peptides in the transmembrane (TM) state have one terminus at each of the two membrane interfaces, while peptides in the surface-bound (S) state have both termini in the same membrane interface. This allows plotting the state transitions from the analysis of the peptide termini position along the membrane normal ( a ). Knowledge of the state as a function of simulation time allows direct determination of the S and TM population averages, as well as analysis of state lifetimes, transition rates and related kinetics. The populations and associated free energies are given in Table 1 . ( c ) Plots of the block-averaged TM-state propensity against the simulation time shows that the systems require at least 3 μs for full convergence. The equivalent kinetics for the L 7 RL 7 CHARMM simulation shows similar Δ G , but much slower kinetics (see Supplementary Fig. 5 ). 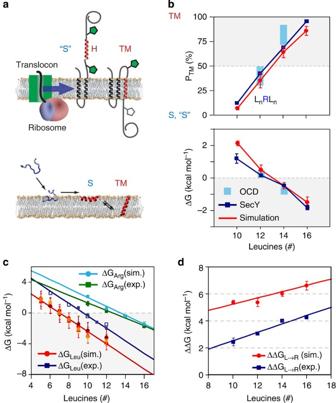Figure 4: Summary of insertion LnRLnpropensity data and comparison with L2ndata. The error bars are given by ±σ, whereσis the s.d. of the mean. (a) Schematic comparison of translocon-guided insertion (upper panel) with simulated spontaneous partitioning (lower panel). (b) Whole-peptide partitioning propensity (PTM) and insertion free energy (ΔG) as a function of the total number of leucines of the LnRLnpeptides. Data in red circles show the results from the monomeric partitioning simulations (cf.Table 1). The blue squares show the experimental apparent insertion propensities measured from the Sec61 translocon assay, and the light blue data points show the results from the oriented circular dichroism (OCD) experiments, which could only be obtained for two peptides: L6RL6(PTM≈30–50%, ΔG≈0–0.5 kcal mol−1) and L7RL7(PTM≈70–90%, ΔG≈−0.5 to −1.1 kcal mol−1). The structure of the singly glycosylated species is a TM helix, the structure and configuration of the doubly glycosylated peptide variant (corresponding to the S state) is not known, and is thus denoted by “S”. (c) Comparison of polyleucine data with LnRLndata. The previously determined free energy of peptide insertion ΔGas a function of the total number of leucine residues shows a ~2 kcal mol−1offset between translocon experimental values (blue) and simulation-derived values (red) for pure polyleucine sequences13,14. However, for polyleucine sequences carrying a central arginine, the translocon-based experimental free energies (green) and simulation-derived partitioning free energies (light blue) are almost identical. (d) The free-energy penalty of replacing the central leucine with an arginine residue (ΔΔGL→R) is calculated by subtracting the ΔGof the equivalent polyleucine (Ln) peptide from the ΔGof the LnRLnpeptide (for example, L11for L5RL5). The difference between the experimental (blue) and simulation (red) ΔΔGis almost entirely due to the constant free-energy offset of the polyleucine peptides, with a small contribution due to differing slopes of the arginine-containing peptides. Due to deeper burial of the guanidinium side chain for longer peptides, the penalty of swapping a leucine with an arginine at the center of a polyleucine segment increases linearly with peptide length (seeFig. 3;Supplementary Table 2). Full size image Figure 4: Summary of insertion L n RL n propensity data and comparison with L2 n data. The error bars are given by ± σ , where σ is the s.d. of the mean. ( a ) Schematic comparison of translocon-guided insertion (upper panel) with simulated spontaneous partitioning (lower panel). ( b ) Whole-peptide partitioning propensity ( P TM ) and insertion free energy (Δ G ) as a function of the total number of leucines of the L n RL n peptides. Data in red circles show the results from the monomeric partitioning simulations ( cf. Table 1 ). The blue squares show the experimental apparent insertion propensities measured from the Sec61 translocon assay, and the light blue data points show the results from the oriented circular dichroism (OCD) experiments, which could only be obtained for two peptides: L 6 RL 6 (P TM ≈30–50%, Δ G ≈0–0.5 kcal mol −1 ) and L 7 RL 7 (P TM ≈70–90%, Δ G ≈−0.5 to −1.1 kcal mol −1 ). The structure of the singly glycosylated species is a TM helix, the structure and configuration of the doubly glycosylated peptide variant (corresponding to the S state) is not known, and is thus denoted by “S”. ( c ) Comparison of polyleucine data with L n RL n data. The previously determined free energy of peptide insertion Δ G as a function of the total number of leucine residues shows a ~2 kcal mol −1 offset between translocon experimental values (blue) and simulation-derived values (red) for pure polyleucine sequences [13] , [14] . However, for polyleucine sequences carrying a central arginine, the translocon-based experimental free energies (green) and simulation-derived partitioning free energies (light blue) are almost identical. ( d ) The free-energy penalty of replacing the central leucine with an arginine residue (ΔΔ G L→R ) is calculated by subtracting the Δ G of the equivalent polyleucine (L n ) peptide from the Δ G of the L n RL n peptide (for example, L 11 for L 5 RL 5 ). The difference between the experimental (blue) and simulation (red) ΔΔ G is almost entirely due to the constant free-energy offset of the polyleucine peptides, with a small contribution due to differing slopes of the arginine-containing peptides. Due to deeper burial of the guanidinium side chain for longer peptides, the penalty of swapping a leucine with an arginine at the center of a polyleucine segment increases linearly with peptide length (see Fig. 3 ; Supplementary Table 2 ). Full size image The partitioning equilibrium can be summarized in a peptide-tilt versus insertion-depth free-energy surface ( Supplementary Fig. 8 ). The data confirm that the equilibrium is between surface-bound and TM configurations for all peptides. Separation of the configurational ensemble into equilibrium states can be achieved by tracking the motion of the peptide termini along the membrane normal over the course of the simulation. Figure 3 demonstrates that this approach separates a TM configuration (where each bilayer interface hosts exactly one peptide terminus) from a surface-bound one (where one interface harbours both termini). Apart from allowing an accurate quantification of the S- and TM-state populations, this analysis allows calculation of kinetic properties such as the number of transitions and the average lifetimes of the states. All thermodynamic and kinetic data derived from Fig. 3 are summarized in Table 1 , revealing a large number of equilibrium transitions between the S and TM states for all peptides. Configurational equilibria in molecular dynamics simulations rely crucially on accurate force field parameters. To exclude a force field dependency of the results, the L 7 RL 7 peptide simulation was repeated using the CHARMM force field (see Methods). This simulation showed a slightly more-helical and less-flexible peptide ( Supplementary Fig. 9 ). The kinetics were sevenfold slower than for the equivalent OPLS force field simulation, but resulted in a very similar insertion free energy ( Table 1 ). The difference in kinetics between the OPLS and CHARMM simulations is most likely due to the united-atom (OPLS) versus all-atom (CHARMM) nature of the lipid force fields [35] , [36] ; the protein force field was all-atom in both cases. For accurate determination of thermodynamic and kinetic quantities from folding-partitioning simulations, all thermally accessible states of the system must be fully sampled. Furthermore, great care must be taken to check that the resulting thermodynamic ensemble is fully converged and that the relative populations of the states present at equilibriums have stabilized at their equilibrium values. Tracking the running average of the TM-state propensity ( P TM ) shows that at least 3 μs are required for convergence ( Fig. 3c ). Population averages derived from a higher number of transitions between states are more reliable. Because the rate of transitions between states decline exponentially with increasing free-energy differences, the L 6 RL 6 and L 7 RL 7 peptides have the most reliable free energies ( Supplementary Fig. 10 ). Faster convergence of the thermodynamic equilibrium was achieved when the simulation temperature was elevated to 140 °C. We have previously shown that such high temperatures do not affect the thermodynamic equilibrium, because TM helices are highly stable against thermal denaturation due to the large penalty associated with breaking a peptide hydrogen bond in the hydrophobic membrane interior [13] and the decreased aqueous solubility of hydrophobic molecules at elevated temperatures. Consequently, the conformational ensemble of the peptide does not change measurably with temperature. We experimentally verified the thermostability of the peptides embedded in POPC vesicles using SRCD spectroscopy, with essentially no unfolding detected at temperatures up to 85 °C (see Supplementary Fig. 11 ). To verify that the partitioning behaves similarly above the boiling point, we carried out a 6-μs control simulation of L 6 RL 6 at 90 °C. The results show that the insertion propensity P TM =29.9±24.4 (s.d.) at 90 °C is similar to the 140 °C system ( P TM =35.3±7.6 (s.d.)) (see Table 1 ). However, the much smaller number of transitions at the lower temperature resulted in large errors and poor convergence (see Supplementary Fig. 10 ). We estimate that even at 90 °C the simulation would have to be extended by roughly an order of magnitude to achieve the same level of convergence as the 140-°C system. Figure 4 compares the propensity P TM and free energy Δ G TM of TM insertion obtained from the simulations and experiments. Although the OSRCD measurements could only provide estimates of the orientation state population for L 6 RL 6 and L 7 RL 7 , the general agreement between all methods is remarkable. The results suggest that 14 or more leucine residues are sufficient for favourable TM insertion of a hydrophobic polyleucine segment containing a central arginine. We have previously determined the transfer free energies of polyleucine peptides using both folding-partitioning simulations as well as the translocon assay described above [13] , [14] . The contribution of the added arginine side chain to the transfer free energies of the peptides can be estimated by subtracting the transfer free energy of the corresponding polyleucine segments. The analysis reveals that replacing a leucine with an arginine residue at the center of a polyleucine segment results in a free-energy penalty that rises linearly with the length of the peptide ( Fig. 4b ; Supplementary Table 2 ). The linear rise occurs because longer peptides result in deeper burial of the guanidinium group ( Supplementary Fig. 6 ). For translocon partitioning, the free-energy penalty rises from 2.4 kcal mol −1 for replacing the central leucine of L 11 with an arginine, to 4.3 kcal mol −1 for L 17 . Swapping the central leucine with an arginine is more costly in the simulations, with a penalty of 5.4 kcal mol −1 for L 11 and 6.8 kcal mol −1 for L 17 . The discrepancy between the experimental and simulation data seems exclusively due to the constant offset of 2 kcal mol −1 observed between simulation- and translocon-derived insertion free energies of pure polyleucine peptides ( Supplementary Table 2 ). Overall, the free energy penalty for burial of a charged guanidinium group at the heart of a hydrophobic membrane-spanning segment is moderate and consistent with earlier translocon data, which measured only minor energetic penalties [9] , [10] . The present approach suggests that using simulations to provide an atomic-detail picture of the system can provide complementary insights for experimental measurements that are not possible to achieve with either approach individually. In the present case, the experimental OSRCD and translocon measurements provide time-averaged structural and energetic equilibrium data, while the simulations report the peptide configurations and dynamics in the bilayer that give rise to these thermodynamic measurements. This knowledge of the equilibrium states, between which the equilibrium is measured, is vital for the development of accurate models. The reasons for the offset of the polyleucine partitioning free energies, especially in light of the excellent agreement between translocon and simulation data for the arginine-containing peptides presented here, are currently not clear. One interpretation might be that a charge inside the hydrophobic segment might give the translocon less leeway than a pure hydrophobic segment. It has been suggested that arginine insertion into bilayers is favourable due to dimerization [25] . Although the simulation data show that the peptides insert efficiently as monomers, this does not preclude a further lowering of the insertion free energy for dimeric TM configurations, which might reintroduce the offset between translocon and simulation data observed for pure polyleucine peptides. To test the dimerization hypothesis, we performed a simulation with two L 6 RL 6 peptides in the same bilayer patch. The results, summarized in Fig. 5 , show that although the peptides meet many times during the course of the simulation, and occasionally form a common defect in the membrane, aggregates have a short lifetime. We conclude that the two peptides generally partition independently of each other, particularly because the insertion propensity P TM =30.2±7.9% is similar for both peptides and close to the value observed for the single peptide simulation (35.3±7.6%). Furthermore, the two-peptide data suggest that partitioning of the peptides is monomeric, with no further energetic gain through aggregate formation, although it should be noted that the timescale of the simulations might be too short to capture the formation of a stable aggregate. 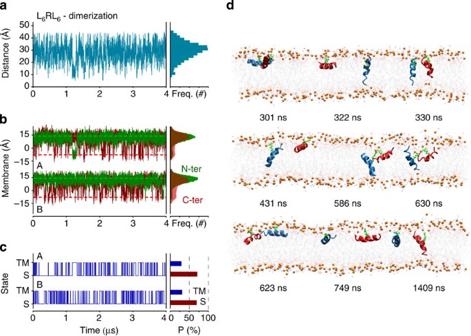Figure 5: Equilibrium simulation (4 μs) of two L6RL6peptides to test for dimerization. (a) Analysis of the inter-arginine distance. The figure plots the distance between the CZ atoms of the two guanidinium side chains. The figure shows that the peptides diffuse randomly, independent of each other and any aggregate formation is short-lived, with the longest observed contact lasting ~90 ns (at 1.17 μs). (b) Analysis of the positions of the peptide N termini (green) and C termini (red) along the membrane normal reveals that each peptide partitions independently of the other. (c) The state transitions from the analysis of the peptide termini position along the membrane normal (b) show that both peptides have similar S- and TM-state populations and associated free energies (seeTable 1). (d) Snapshots of the dimer simulation show independent partitioning of the peptides with occasional random collision, no stable aggregate formation was observed. See movies LnRLn_dimer_side.mov and LnRLn_dimer_top.mov in onlineSupplementary Information. Figure 5: Equilibrium simulation (4 μs) of two L 6 RL 6 peptides to test for dimerization. ( a ) Analysis of the inter-arginine distance. The figure plots the distance between the CZ atoms of the two guanidinium side chains. The figure shows that the peptides diffuse randomly, independent of each other and any aggregate formation is short-lived, with the longest observed contact lasting ~90 ns (at 1.17 μs). ( b ) Analysis of the positions of the peptide N termini (green) and C termini (red) along the membrane normal reveals that each peptide partitions independently of the other. ( c ) The state transitions from the analysis of the peptide termini position along the membrane normal ( b ) show that both peptides have similar S- and TM-state populations and associated free energies (see Table 1 ). ( d ) Snapshots of the dimer simulation show independent partitioning of the peptides with occasional random collision, no stable aggregate formation was observed. See movies LnRLn_dimer_side.mov and LnRLn_dimer_top.mov in online Supplementary Information . Full size image A particularly important observation is that during the simulations the initially unfolded peptides in solution quickly partition into the lipid bilayer interface, never to leave, so that the equilibrium states observed are interfacial and TM. This means that the free energies measured in the simulation are those for transferring the helices from the bilayer interface into and across the bilayer ( Fig. 1b ). The interfacial location is expected from extensive experimental studies of the partitioning of amphipathic peptides, such as melittin [37] , [38] , [39] , [40] . A folded interfacial state is preferred because of the high cost of partitioning peptide bonds into the interface or across the bilayer [2] . The formation of intramolecular hydrogen bonds of α-helices markedly reduces the cost of partitioning, making the folded interfacial state the preferred state, as observed here. There is no reason to believe that interfacial folding is not also important biologically. Unless the translocon completely isolates nascent helices emerging from the ribosome, helix–interface interactions are likely to be important in translocon-guided insertion. In fact, we know that the translocon–ribosome connection is quite exposed to the cytoplasm [41] , [42] , [43] , [44] . One might thus speculate that the membrane interface in the vicinity of the translocon plays an important role in translocon-guided TM helix insertion. Peptide designs Translocon experiments. The flanks of the L n RL n hydrophobic segment were extended to include –GGPG– at the N-terminal end and –GPGG– at the C-terminal end to insulate the hydrophobic segment from the surrounding LepB carrier protein. Synthetic experiments . Acetyl-GWL n −1 -R-L n G-amide ( n =5–8). The N-terminal leucine of each peptide was replaced with a tryptophan to aid purification and quantification of peptide concentration for the spectroscopic experiments, exploiting the average molar extinction coefficient of ε =5,600 M −1 cm −1 of the tryptophan indole moiety at 280 nm [45] . Computational experiments . Ace-GL n -R-L n G-ame ( n =5–8). The N- and C termini were acetylated (ace) and amidated (ame), respectively, to reduce the kinetic barrier associated with TM insertion of the peptide, which involves transport of a polar peptide terminus across the hydrophobic membrane core. Sec61 translocon insertion assay Enzymes and chemicals . Unless stated otherwise, all chemicals were from Sigma-Aldrich (St Louis, MO, USA). Oligonucleotides were purchased from MWG Biotech AG (Ebersberg, Germany). Pfu Turbo DNA polymerase was purchased from Agilent Technologies. All other enzymes were from Fermentas. The plasmid pGEM-1 and the TNT SP6 Transcription/Translation System were from Promega. [ 35 S]Met was from PerkinElmer. DNA manipulations . All LepB constructs used carried one acceptor site for N-linked glycosylation in positions 97–99 (Asn-Ser-Thr) and the naturally present acceptor site in positions 215–217 (Asn-Glu-Thr). LepB constructs encoding H-segments with different numbers of leucines were generated by modifying the lepB gene in the pGEM-1 vector containing SpeI and KpnI restriction sites [9] . Double-stranded oligonucleotides encoding H-segments with GGPG/GPGG flanks including either N-terminally a SpeI or C-terminally a KpnI restriction site were created by annealing two pairs of complementary oligonucleotides with overlapping overhangs. All sequences encoding different H-segments and the pGEM-1 vector were digested with SpeI and KpnI, followed by insertion of the H-segments into the cut vector by ligation. Oligonucleotides were diluted to a concentration of 20 μM. Twenty microlitres of each forward and reverse complementary segment (sample 1: forward1+reverse1; sample 2: forward2+reverse2) were mixed with 4.4 μl annealing oligonucleotide buffer (20 mM Tris-HCl pH 7.4, 20 mM MgCl 2 and 500 mM NaCl) and heated at 85 °C for 10 min. Samples were left in the heating block until the temperature was <30 °C. Twenty microlitres each of the annealed samples 1 and 2 were mixed and heated at 65 °C for 5 min. Samples were left in the heating block until the temperature was <30 °C. The annealed H-segment was ligated into the cut vector overnight at 16 °C followed by transformation. All inserts and mutagenesis were confirmed by sequencing of plasmid DNA at Eurofins MWG Operon (Ebersberg, Germany). Oligonucleotide sequences were as follows: L 5 RL 5 : forward first part: 5′-P-CTAGTGGTGGTCCTGGActgcttctgcttctg cgt ctg-3′; forward second part: 5′-P-cttctgcttctgGGACCTGGTGGGGTAC-3′; reverse first part: 5′-P-cagaagcagTCCAGGACCACCA-3′; reverse second part: 5′-P-CCCACCAGGTCCcagaagcagaagcagacgcagaag-3′. L 6 RL 6 : forward first part: 5′-P-CTAGTGGTGGTCCTGGActgctgcttctgcttctg cgt ctg-3′; forward second part: 5′-P-cttctgcttctgctgGGACCTGGTGGGGTAC-3′; reverse first part: 5′-P-cagaagcagcagTCCAGGACCACCA-3′; reverse second part: 5′-P-CCCACCAGGTCCcagcagaagcagaagcagacgcagaag-3′. L 7 RL 7 : forward first part: 5′-P-CTAGTGGTGGTCCTGGActgctgctgcttctgcttctg cgt ctg-3′; forward second part: 5′-P-cttctgcttctgctgctgGGACCTGGTGGGGTAC-3′; reverse first part: 5′-P-cagaagcagcagcagTCCAGGACCACCA-3′; reverse second part: 5′-P-CCCACCAGGTCCcagcagcagaagcagaagcagacgcagaag-3′. L 8 RL 8 : forward first part:5′-P-CTAGTGGTGGTCCTGGActgctgctgctgcttctgcttctg cgt ctg-3′; forward second part: 5′-P-cttctgcttctgctgctgctgGGACCTGGTGGGGTAC-3′; reverse first part: 5′-P-cagaagcagcagcagcagTCCAGGACCACCA-3′; reverse second part: 5′-P-CCCACCAGGTCCcagcagcagcagaagcagaagcagacgcagaag-3′. L 9 RL 9 : forward first part: 5′-P-CTAGTGGTGGTCCTGGActgctgctgctgctgcttctgcttctg cgt ctg-3′; forward second part: 5′-P-cttctgcttctgctgctgctgctgGGACCTGGTGGGGTAC-3′; reverse first part: 5′-P-cagaagcagcagcagcagcagTCCAGGACCACCA-3′; reverse second part: 5′-P-CCCACCAGGTCCcagcagcagcagcagaagcagaagcagacgcagaag-3′. Expression in vitro . Constructs cloned in pGEM-1 were transcribed and translated in the TNT Quick coupled transcription/translation system. One microgram of DNA template, 1 μl of [ 35 S]Met (10 μCi; 1 Ci=37 GBq), 1 μl of RNasin, 1 μl of a mixture of all 20 natural amino acids minus methionine and 1 μl of dog pancreas RMs were mixed with 9 μl of TNT lysate mix, and samples were incubated for 90 min at 30 °C. The sample was mixed with SDS sample buffer [10] and incubated at 90 °C for 5 min before loading on a 12% SDS/polyacrylamide gel. Proteins bands were visualized in a Fuji FLA-3000 phosphoimager (Fujifilm, Tokyo, Japan). The Image Gauge V 4.23 software (Fujifilm) was used to generate a two-dimensional intensity profile of each gel lane, and the multi-Gaussian fit program from the Qtiplot software package ( www.qtiplot.ro ) was used to calculate the peak areas of the protein bands. An apparent equilibrium constant between the membrane-integrated and non-integrated forms was calculated as: K app = f 1g / f 2g , where f 1g is the fraction of singly glycosylated LepB molecules and f 2g is the fraction of doubly glycosylated LepB molecules. The results were then converted to apparent free energies, Δ G app =− RT ln K app . Synthetic peptide experiments Synthesis and purification . All peptides were solid-state synthesized on amide resins using standard FMOC/HBTU chemistry, purified using reverse-phase high-pressure liquid chromatography, and quantified using mass spectroscopy. The peptides were injected in 100% formic acid and separated using C4-C18 columns with acetonitrile–water gradients (0.1% trifluoroacetic acid) and lyophilized. Sample preparation . Samples were prepared by mixing stock solutions of peptide in trifluorethanol and POPC lipids in chloroform (Avanti Polar Lipids, Alabaster, AL, USA). The mixture was desolvated under a stream of nitrogen with subsequent overnight incubation under vacuum to remove solvent. Vesicles were prepared by rehydrating dry peptide/lipid films in distilled water at room temperature. Vesicles were prepared by extrusion through membranes with 200-nm pores. The peptide concentration in all samples was 30 μM, and the molar peptide/lipid ratio was 1/100. Stacked lipid bilayers were prepared by dissolving peptide/lipid mixtures in trifluorethanol and application to Suprasil quartz slides at peptide/lipid ratios of 1/20–1/200, and hydrating them in a specially designed sample chamber [46] . The peptide concentrations of all samples were 1 mg ml −1 . SRCD spectroscopy . Circular dichroism spectra were collected at the CD12 beamline at ANKA (Karlsruhe, Germany), the CD1 beamline at ISA (Århus, Denmark), and beamline 4B8 at the Beijing Synchrotron Radiation Facility (China) [47] . OSRCD spectra were collected for eight rotation angles of the quartz substrate around the axis of the beam and averaged to limit linear dichroism effects. Data were collected from 280 to 180 nm at 1 nm intervals and 1 nm bandwidth. The response time was 2–4 s at each wavelength and each measurement was an average of four scans. Temperature was controlled with a Peltier device, and varied between 20 and 85 °C in 5 °C steps. Samples were equilibrated for at least 5 min at each temperature before data collection. All spectra were corrected for background by subtracting the corresponding vesicle-only spectrum measured over the same temperature range. Spectral and metadata deposited in the Protein Circular Dichroism Data Bank will be released upon publication. Molecular dynamics simulations Simulations were performed and analysed with Gromacs 4.5 ( www.gromacs.org ) [48] and hippo beta ( www.biowerkzeug.com ), using the OPLS all-atom protein force field [49] in conjunction with the TIP3P water model [50] . OPLS united-atom lipid parameters for POPC were taken from Ulmschneider et al. [35] Control simulations were carried out with the CHARMM27 protein, and CHARMM36 lipid force fields, with TIP3P water. Electrostatic interactions were computed using Particle mesh Ewald (PME) algorithm. A cutoff of 10 Å was used for van der Waals interactions. Bonds involving hydrogen atoms were constrained using LINCS [51] . The integration time-step was 2 fs and neighbour lists were updated every five steps. All simulations were performed in the isothermal isobaric ensemble with constant particle number (NpT), without any restraints or biasing potentials. Water, lipids and the protein were each coupled separately to a heat bath with time constant τ T =0.1 ps using weak temperature coupling [52] . Atmospheric pressure of 1 bar was maintained [53] using weak semi-isotropic pressure coupling with compressibility κ z = κ xy =4.6 × 10 –5 bar –1 and time constant τ P =1 ps. Before production runs all systems were equilibrated for 2–10 ns. Free-energy surfaces The free-energy surfaces were calculated as a function of the peptide’s center-of-mass position along the membrane normal and the tilt angle. A two-dimensional normalized histogram was calculated over the equilibrium phase of the simulations. Each ‘bin’ contains the probability p i of finding the peptide in state i. For a system in thermodynamic equilibrium, the change in free energy on going from one state to another is given by where R is the ideal gas constant and T is the temperature. The relative free energy was calculated for each bin, and the minimum was shifted to zero. Insertion propensity and free energy The insertion propensity P TM = f TM /( f TM + f S ) of each peptide is calculated as the probability of the peptide being in the TM state. To distinguish the TM state from the S conformations, the position of the peptide termini along the membrane normal was tracked. The insertion free energy, or ‘free energy of partitioning’ can be directly calculated from the TM-state propensity using Helicity The helicities of the peptides were calculated for each residue, and then averaged over the complete sequence. A residue is considered helical if its backbone dihedral angles are within ±40° from the ideal α-helical values (Φ=–57°, Ψ=–47°). Error estimates In all figures, we determined error bar estimates by dividing the simulations into a series of 10 blocks of equal length, and then performing averaging for each block. The error bars are given by ± σ , where σ is the s.d. of the mean, that is, the s.d. of the individual block averages with respect to the overall average. How to cite this article : Ulmschneider, M. B. et al. Spontaneous transmembrane helix insertion thermodynamically mimics translocon-guided insertion. Nat. Commun. 5:4863 doi: 10.1038/ncomms5863 (2014).